Covalency of hydrogen bonds in liquid water can be probed by proton nuclear magnetic resonance experiments The concept of covalency is widely used to describe the nature of intermolecular bonds, to explain their spectroscopic features and to rationalize their chemical behaviour. Unfortunately, the degree of covalency of an intermolecular bond cannot be directly measured in an experiment. Here we established a simple quantitative relationship between the calculated covalency of hydrogen bonds in liquid water and the anisotropy of the proton magnetic shielding tensor that can be measured experimentally. This relationship enabled us to quantify the degree of covalency of hydrogen bonds in liquid water using the experimentally measured anisotropy. We estimated that the amount of electron density transferred between molecules is on the order of 10 m while the stabilization energy due to this charge transfer is ∼ 15 kJ mol −1 . The physical insight into the fundamental nature of hydrogen bonding provided in this work will facilitate new studies of intermolecular bonding in a variety of molecular systems. From its early days, NMR spectroscopy has been instrumental in the study of liquid water [1] , [2] . The magnetic shielding tensor, which relates secondary induced electronic magnetic fields to an external static magnetic field, is at the heart of NMR spectroscopy. The shielding tensor is characterized by the three components in the principal axes frame σ X ≤ σ Y ≤ σ Z or, alternatively, by the isotropic part σ iso = ( σ X + σ Y + σ Z ), the anisotropy Δ= σ Z − σ iso , and the asymmetry η = ( σ Y − σ X ) [3] . However, because of the random orientation and motion of molecules in the liquid phase, only the isotropic part of the tensor can be directly measured by experiment. Nevertheless, even the isotropic 1 H shielding can provide valuable information: it has been long established that σ iso decreases on the formation of hydrogen bonds (HBs) [4] , [5] , [6] . A quantitative investigation between the other components of the shielding tensor and the HB geometry in liquid water [7] , [8] and small cluster models [4] , [9] , [10] has been made possible by advances in electronic structure theory [11] , [12] , [13] , [14] , [15] , [16] . Moreover, a recently reported elegant experimental approach has allowed the indirect measurement of the 1 H shielding anisotropy in liquid water via its contribution to spin relaxation rates [17] . Combined with first principles calculations, the new experimental data [8] have underscored previous findings that some of the tensor components are more sensitive to HB interactions than the average σ iso (refs 4 , 18 ). In this work, we reveal a quantitative relationship between the calculated components of the 1 H magnetic shielding tensor and the degree of covalency of HBs in liquid water [19] , [20] . The covalent component of intermolecular bonds is commonly defined as the strength of donor–acceptor orbital interactions between molecules [21] . Covalency, like many other individual fundamental mode of binding (for example, frozen electrostatics, polarization), cannot be measured, even in principle, by experiment; only the total strength of binding is measurable. Nevertheless, similar to various other unmeasurable auxiliary concepts (for example, wave function in quantum mechanics), covalency is a fundamental, theoretically well defined and physically meaningful quantity that is widely used by chemists to investigate the nature of intermolecular bonding. Furthermore, it is widely accepted that donor–acceptor interactions between molecules in liquid water affect its directly measurable structural, spectroscopic and chemical properties. Decomposition analysis and NMR shielding tensor To quantify the strength of covalent interactions in a HB, we employed the decomposition analysis for condensed phase systems based on absolutely localized molecular orbitals (ALMO DA) [21] , [22] within Kohn–Sham density functional theory [23] . The ALMO DA makes this feat possible by first filtering out frozen electrostatic and polarization effects from the total many-body intermolecular binding energy, and then splitting the remaining covalent component into two-body terms, each corresponding to an individual HB. The ALMO approach allows to define two scales to measure the strength of covalent interactions: the amount of electron density transferred from the occupied orbitals on molecule A to the virtual orbitals on molecule B (Δ Q A→B ), and the energetic stabilization due to this charge transfer (Δ E A→B ). These two-body terms are obtained self-consistently and include cooperativity effects, which are essential for a correct description of the HB network in liquid water [24] , [25] , [26] , [27] . 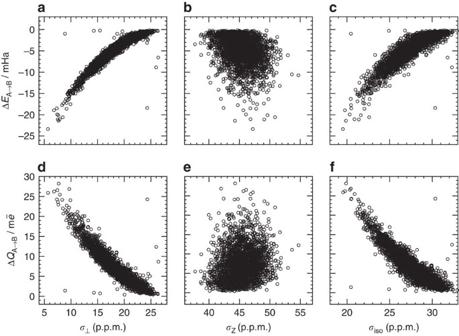Figure 1: Relationship between the electronic descriptors and NMR characteristics of HBs. ΔEA→Band ΔQA→Bas a function ofσ⊥,σZandσiso, respectively. All ensemble averaged components of the NMR shielding tensor ( Table 1 ), geometric and ALMO DA descriptors of HBs were calculated from density functional theory-based ab initio molecular dynamics (MD) simulations performed to represent liquid water at ambient conditions (see Methods for details). The computed values are close to the experimentally measured absolute shielding values at 27 °C ( σ iso =25.7 p.p.m. and Δ=18.3 p.p.m., respectively) [17] . We followed the common practice of denoting the average of σ X and σ Y components of the axially nearly symmetric NMR tensors ( η ≈0) as the perpendicular shielding component σ ⊥ . It is easy to see that σ ⊥ is directly related to the anisotropy: σ ⊥ = σ iso − . Table 1 Calculated ensemble averaged shielding tensor components in p.p.m. for liquid water at ambient conditions. Full size table Correlation between σ components, HB covalency and geometry Figure 1a,d show that σ ⊥ exhibits a striking correlation with the strength of electron density transfer as measured on both charge and energy scales. By comparison, the correlation between σ iso and the strength of charge transfer ( Fig. 1c,f ) is weaker, because σ iso is just the strongly correlated σ ⊥ component plus the noise from σ Z ( Fig. 1b,e ). Figure 1: Relationship between the electronic descriptors and NMR characteristics of HBs. Δ E A→B and Δ Q A→B as a function of σ ⊥ , σ Z and σ iso , respectively. Full size image The presence of the scattered points in Fig. 1 that do not follow the general trend is a manifestation of the complex nature of the HB network, in which some hydrogen atoms do not form HBs and some interact strongly with more than one electron donor. Describing such configurations in detail is beyond the scope of the present work and will be presented elsewhere. Here we just would like to note that including or excluding the outliers does not change our statistical results, models or conclusions significantly (see Methods). To obtain a more comprehensive view on HBs in liquid water we collected information on the correlation between electronic, NMR and geometric descriptors into a single matrix shown in Fig. 2 . In addition to the key relationship established above, the correlation matrix clearly shows the well-known relationship between the HB length and σ iso . However, we found that the correlation of the HB length and σ ⊥ is stronger. As in the case of the electronic descriptors, the correlation between the HB length and σ iso is merely a manifestation of the underlying strong correlation with σ ⊥ plus a noisy contribution from σ Z . 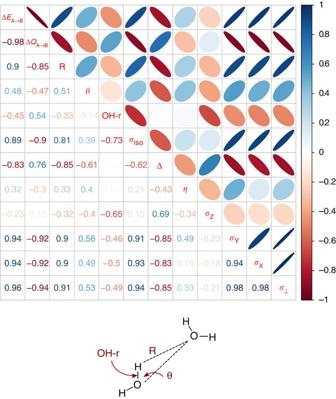Figure 2: Correlation matrix between the1H shielding tensor components and HB descriptors. The descriptors are shown on the main diagonal. The lower part of the matrix gives numerical values of the Pearson correlation coefficientrbetween a pair of variables. The upper part above the diagonal presents a symbolic representation of the same correlation: ellipses represent different degrees of correlation ranging fromr=1 (straight line) tor=0 (perfect circle). The geometric descriptors are illustrated on the water dimer at the bottom, where OH-r is the covalent O-H bond length andRthe HB length, whileθis the HB angle. Figure 2: Correlation matrix between the 1 H shielding tensor components and HB descriptors. The descriptors are shown on the main diagonal. The lower part of the matrix gives numerical values of the Pearson correlation coefficient r between a pair of variables. The upper part above the diagonal presents a symbolic representation of the same correlation: ellipses represent different degrees of correlation ranging from r =1 (straight line) to r =0 (perfect circle). The geometric descriptors are illustrated on the water dimer at the bottom, where OH-r is the covalent O-H bond length and R the HB length, while θ is the HB angle. Full size image Δ Q A→B and Δ E A→B are also strongly correlated with the HB length, even though this correlation is somewhat weaker than that with σ ⊥ because the HB length alone is insufficient to characterize a HB (that is, other geometric descriptors, such as the HB angle, should be taken into account). We note that no correlations were found for the electron transfer terms where the water molecule bearing the shielding tensor acts as an electron donor. This shows that the 1 H shielding tensor is insensitive to electron transfer from the lone pairs of its own water molecule. There is no significant correlation of the HB angle with any individual shielding tensor component, except for a rather weak correlation with Δ. The HB angle alone does not appear to influence electronic terms either, in agreement with the insensitivity of Δ Q A→B and Δ E A→B to intermolecular rotations in water dimer [28] . In addition to studying the shape of the shielding ellipsoid, we also examined its orientation relative to the water molecule. As in previous studies [29] , our simulations showed that the longest Z axis of the tensor points along the covalent O—H bond: the mean deviation angle between the longest axis and the covalent O—H bond is only 5±3° ( Fig. 3 , top). Moreover, despite the very low value of η , we find that the two short axes still exhibit a distinct spatial preference: the shortest X axis is normal to the plane of the water molecule, whereas the intermediate Y axis is coplanar with the molecule ( Fig. 3 , bottom). In other words, the shielding tensor is rigidly fixed to the water molecule. Previous reports have shown that the only non-zero off-diagonal elements of the shielding tensor are σ yz and σ zy in the Eckart frame [7] , [30] . This is consistent with our finding, as the transformation from the principal axes frame to the Eckart frame is merely a rotation around the X axis. 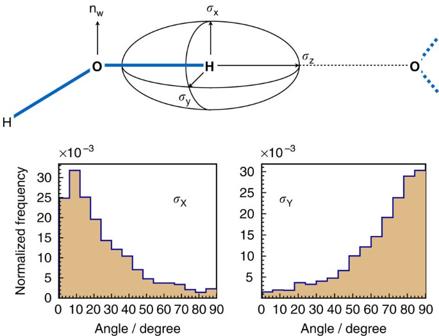Figure 3: Spatial orienation of the1H shielding tensor relative to the HB geometry. The1H shielding tensor ellipsoid is rigidly fixed to the molecular frame of the HB donating water molecule. The longest axis of the ellipsoid (σZ) always points along the HB. The angle between the normal to the water molecular plane (nw) andσXandσYshow that the former is parallel to nw, while the latter is orthogonal to it. Figure 3: Spatial orienation of the 1 H shielding tensor relative to the HB geometry. The 1 H shielding tensor ellipsoid is rigidly fixed to the molecular frame of the HB donating water molecule. The longest axis of the ellipsoid ( σ Z ) always points along the HB. The angle between the normal to the water molecular plane (n w ) and σ X and σ Y show that the former is parallel to n w , while the latter is orthogonal to it. Full size image Linear model that relates σ ⊥ to the covalency of HBs The physical basis underlying the correlation between the electronic and NMR terms ( Fig. 1 ) can be understood by considering the dependence of both of these quantities on the HB length R . We found that σ x and σ y decrease linearly with R −3 over the entire HB length range in liquid water (see Supplementary Fig. 1 ). This strong negative correlation implies that the induced magnetic field from the electron donor molecule (a schematic depiction is given in Supplementary Fig. 2 ) is the major contributor to deshielding in the plane orthogonal to the HB—it accounts for 88% of the variance in σ ⊥ . The inverse cubic dependence also suggests that this field can be accurately represented as that of a magnetic dipole. That is, higher order terms in the multipole expansion ( Supplementary Equation 1 ) are negligible. Thus, the R −3 dependence of σ ⊥ enables one to write: where σ ⊥ ∞ characterizes an HB-free water molecule, and has a value of 33.7 p.p.m. as obtained by linearly extrapolating σ ⊥ to R −3 =0. The strength of donor–acceptor interactions between molecules decreases with the tails of the orbitals, that is, exponentially with distance [21] The combination of the two equations predicts the following relationship between the charge-transfer term and perpendicular component of the NMR shielding tensor: where γ Q =− β Q α 1/3 is the dimensionless proportionality constant. A similar relationship can be written for the energy scale with β E , γ E , λ E as parameters. Indeed, plotting both sides of equation (3) reveals clear linear trends ( Fig. 4 ) with a Pearson coefficient of −0.94 for Δ E A→B and −0.92 for Δ Q A→B . The values of the parameters that represent the best fit of the simulation data are λ Q =270.6 m , λ E =579.4 mHa, γ Q =− 19.86 and γ E =−24.07, respectively. It is worth noting that the λ coefficients should not be interpreted as the limiting values for R →0, but rather as statistical coefficients that best fit the linear trend over its limited range of validity. 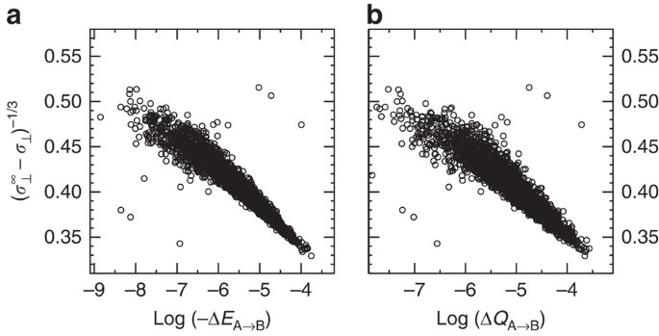Figure 4: The derived linear model relatingσ⊥to the electronic descriptors as obtained by ALMO DA. Dependence between (σ⊥∞−σ⊥)−1/3and: (a) log(−ΔEA→B), (b) log(ΔQA→B). Figure 4: The derived linear model relating σ ⊥ to the electronic descriptors as obtained by ALMO DA. Dependence between ( σ ⊥ ∞ − σ ⊥ ) −1/3 and: ( a ) log(−Δ E A→B ), ( b ) log(Δ Q A→B ). Full size image While σ ⊥ shows the strong R −3 dependence, the weak correlation between σ Z and R −3 ( Supplementary Fig. 1 ) indicates that the change in σ Z results from the factors other than the dipolar field of the electron donor molecule. We found that a satisfactory regression model capable of predicting the behaviour of σ Z should include at least three predictor variables: R −3 , the HB angle θ and the covalent O—H bond length OH-r. The standardized regression coefficients of this model ( Supplementary Table 1 ) show that R −3 and OH-r give opposite contributions to σ Z largely cancelling each other out. The established quantitative dependence between σ ⊥ and the strength of intermolecular donor–acceptor bonding has one important implication: since σ ⊥ can now be measured experimentally in liquids [17] , our model represents an indirect method for probing the covalent component of HBs. Table 2 presents our estimates of Δ E A→B and Δ Q A→B in liquid water based on a linear approximation to the regression model established here and the σ ⊥ measured experimentally at different temperatures [17] ( Supplementary Note 1 for full analysis). As expected, the strength of the covalent component in HBs decreases with increasing temperature as more water molecules form distorted or even broken HBs with their neighbours. Table 2 Estimated average values for Δ E A→B and Δ Q A→B in liquid water at different temperatures. Full size table We would like to emphasize that, unlike population analysis methods (for example, Mulliken, Löwdin), which partition the total electron density between molecules, the ALMO approach measures the reorganization of electron clouds on the formation of a HB [31] . This conceptual advantage of the ALMO method leads to the remarkable result that the fractional electron transfer Δ Q A→B between water molecules in the liquid phase is only a few milli-electrons ( Table 2 ). The reorganization of charge has a well-defined energy given by the Δ E A→B term. Whereas it may seem unusual that so little charge transfer (7–10 m ) can stabilize a HB by 12–18 kJ mol −1 (equivalent to 19 eV per one transferred electron), it is consistent with simple theoretical estimates. Perturbation theory shows that the transfer energy per electron is equal to the energy gap between donating and accepting orbitals [28] . Since the energy gap between the most important donating and accepting orbitals on two molecules lies between 10 and 40 eV (virtual orbitals form almost a continuum of states), a value of 19 eV for the effective donor–acceptor gap is entirely reasonable. To put the estimates of Δ Q A→B into a context, we calculated that 4 m is transferred between molecules in the water dimer if the two molecules are at their equilibrium separation of 2.0 Å. However, Δ Q A→B becomes 7.6 m (that is, significantly closer to the value obtained for the ambient liquid) if the molecules in the dimer are separated only by 1.77 Å—the typical length of a HB in the liquid phase [27] . It is important to note that the timescale of fluctuations in Δ Q A→B and Δ E A→B is the same as the timescale of intermolecular vibrations—hundreds of femtoseconds [22] , [32] , [33] , [34] , which is several orders of magnitude faster than the typical timescale of NMR spectroscopy. This implies that NMR measurements of covalency are capable of yielding only time-averaged values of Δ Q A→B and Δ E A→B . To summarize, we established a simple quantitative relationship between the perpendicular component σ ⊥ of the axially nearly symmetric 1 H magnetic shielding tensor and the degree of covalency of HBs in liquid water. Covalency was defined as the amount of electron density transfer between water molecules and the stabilization energy associated with it. The physical origin of this relationship is the field induced almost entirely by the magnetic dipole located on the neighbouring water molecule involved in the HB. The major implication of our findings is that this relationship provides the calibration necessary to quantify the covalency of HBs experimentally. Recent advancements in measuring σ ⊥ for liquid water [17] enabled us to estimate that the average amount of charge transferred between the molecules on the formation of an average HB is on the order of 10 m , while the corresponding stabilization energy is estimated to be 15 kJ mol −1 . From the practical perspective, using σ ⊥ rather than σ X or σ Y offers an experimental advantage because σ ⊥ can be determined as a linear combination of σ iso and Δ and it is technically easier to measure the latter. In contrast to σ ⊥ , the σ Z component of the shielding tensor exhibits a complex dependence on the local environment around the proton. Its fluctuations cannot be explained only by the magnitude of the induced magnetic fields originating at the proton-accepting water molecule. Therefore, although it is trivial to measure σ iso experimentally, the noisy contribution of σ Z makes it unsuitable for predicting covalency. Second generation Car–Parrinello ab initio MD simulations Ab initio MD simulations of a periodic cubic cell with 128 light water molecules were performed at constant temperature (330 K to mimic nuclear quantum effects in liquid water at ambient conditions [35] ) and density (0.9966, g cm −3 ) using the second generation Car–Parrinello method [36] , [37] . In this approach, the fictitious Newtonian dynamics of the original Car–Parrinello scheme [38] is replaced with an improved coupled electron-ion dynamics that keeps electrons close to the instantaneous electronic ground state without defining a fictitious mass parameter. The superior efficiency originates from the fact that the iterative wave function optimization is fully bypassed. Thus, not even a single diagonalization step is required, while at the same time allowing for integration time steps up to the ionic resonance limit. The energy and forces were computed using the mixed Gaussian-plane waves approach [39] , where the Kohn–Sham orbitals were represented by an accurate triple- ζ basis set with two sets of polarization functions (TZV2P) [40] , while plane-waves with cutoff of 400 Ry were used to represent the charge density. The BLYP exchange-correlation functional plus a damped interatomic potential to account for van der Waals interactions [41] was employed. Previous works have shown that this set-up provides a realistic description of many important structural, dynamical and spectroscopic characteristics of liquid water, including the partial pair correlation functions, self-diffusion and viscosity coefficients, HB lifetime, vibrational spectra and magnetic shielding tensor components [14] , [15] , [27] , [42] , [43] . The system has been equilibrated at constant temperature and density for 30 ps before ten decorrelated snapshots separated by 1 ps were extracted. Computational analysis The ALMO DA was performed for each snapshot using the same computational set-up as in ref. 22 . The magnetic shielding tensors were computed using density functional perturbation theory [14] , [44] , [45] that is based on the all-electron GAPW method [46] , [47] and IGLO-III basis set [48] . All computations were performed using the QUICKSTEP and ALMO modules of the CP2K suite of programmes [49] . To keep our results consistent, we performed sampling over all protons including the outliers that are clearly visible in Figs 1 and 4 . The only exception is the analysis presented in Fig. 2 (supported by Supplementary Fig. 1 and Supplementary Table 1 ). The data presented in Fig. 2 requires computing geometric characteristics of HBs. These characteristics can be computed only for well defined HBs. To define a HB, we used a geometric criterion that was derived from the two-dimensional ( R versus θ ) potential of mean force [43] , [50] . How to cite this article: Elgabarty, H. et al. Covalency of hydrogen bonds in liquid water can be probed by proton nuclear magnetic resonance experiments. Nat. Commun. 6:8318 doi: 10.1038/ncomms9318 (2015).